Genome-wide analysis inDrosophilareveals age-specific effects of SNPs on fitness traits Most organisms exhibit senescence; a decline in physiological function with age. In nature, rates of senescence vary extensively among individuals and this variation has a significant genetic component; however, we know little about the genes underlying senescence. Here we show the first evidence that individual alleles influence fecundity in an age-specific manner and so the genetic basis of natural variation in fecundity changes dramatically with age. We complete a genome-wide association to identify single-nucleotide polymorphisms (SNPs) affecting lifespan and age-specific fecundity using the Drosophila melanogaster Genetic Reference Panel. We identify 1,031 SNPs affecting fecundity and 52 influencing lifespan. Only one SNP is associated with both early- and late-age fecundity. The age-specific effect of candidate genes on fecundity is validated using RNA interference. In addition, there is a dramatic increase in the number of SNPs influencing fecundity with age. This result provides support for the mutation accumulation theory of aging. Senescence, the decline in physiological function with age, is a nearly universal phenomenon that has been of great interest to evolutionary biologists for nearly a century [1] , [2] . A number of studies have demonstrated that senescence has a genetic component, can respond to selection, and that the rate of age-specific decline among individuals and species has a genetic basis [1] , [2] ; however, the genetic basis of natural variation in senescence remains poorly understood. Several studies have used the fruit fly, Drosophila melanogaster , to explore genetic and non-genetic influences on lifespan and senescence. Among the non-genetic factors, Drosophila lifespan can vary in response to changes in larval densities [3] , heat shock, starvation stress, temperature [4] , courtship activity, mating frequency [5] , sex [3] , [6] , [7] , [8] and nutrition [9] , [10] . It is also expected that lifespan is influenced by the contributions of a large number of alleles with small effects [11] , but that the effects of these alleles also depend on genetic background [3] , [7] . Mutagenesis studies have revealed several genes that influence Drosophila lifespan, many of which are in major pathways like the insulin/insulin-like signalling and target of rapamycin pathways [12] . Attempts to identify loci contributing to natural variation in lifespan used quantitative trait locus (QTL) mapping approaches. Several QTL have also been associated with lifespan in Drosophila [3] , [4] , [6] , and a handful of studies have identified candidate genes from within these QTL regions including shuttlecraft (stc,) ms(2)35Ci [13] , Dopa decarboxylase ( Ddc ) [14] and Catsup [15] . Finally, genome-wide association (GWA) studies [8] , mutant screens [7] and expression profiles [16] , [17] , [18] have uncovered several candidate genes and pathways that have important influences on natural variation in the lifespan; however, much remains to be discovered. We still know relatively little about the molecular genetic basis of natural variation in senescence and how alleles contributing to senescence are maintained in a population despite their negative effects on fitness. Fecundity, the number of eggs or offspring produced by an individual, is a key life history trait because it determines the maximum possible number of offspring and so the maximum value of female fitness [19] . Fecundity is heritable both in the lab and in nature, but it is expected to exhibit low levels of variation at early ages because selective pressure is very high for reproductive success at early ages [20] . Fecundity is also an indicator of senescence, declining as age increases [19] , [21] , [22] . Similar to lifespan, fecundity is influenced by a number of environmental factors like nutrition levels [9] , [10] , [23] , temperature [20] , mating frequency [9] and immune status [24] . However, compared with lifespan, much less is known about the genetic basis of natural variation in fecundity. Although some genes have been associated with lifespan and aging, we still have an incomplete understanding of how genetic effects contribute to senescence and how alleles with deleterious effects persist in populations in the face of strong selection to remove them. Recent work has suggested that the genetic basis of complex traits changes with age [19] , [25] , [26] , but this age-specific pattern has not yet been demonstrated at the level of individual single-nucleotide polymorphisms (SNPs). To gain insight into the genetic basis of natural variation in reproduction and lifespan at the molecular genetic level, we measure age-specific and lifetime fecundity together with lifespan in mated females from the Drosophila melanogaster Genetic Reference Panel (DGRP), a set of 192 Drosophila lines derived from nature that have been completely sequenced [8] . We identify a host of candidate SNPs associated with variation in fecundity and lifespan, and we validate a subset of these candidates using RNA interference (RNAi) lines. The number of SNPs influencing fecundity increases dramatically with age, thus supporting the mutation accumulation (MA) theory of senescence. Further, only one SNP appears in our candidate list at both an early age and a late age, which suggests the genetic basis of natural variation influencing fecundity changes dramatically with age. Genetic variation in age-specific fecundity and lifespan We found significant genetic variation in fecundity at all ages examined as well as in lifespan using a mixed-model analysis of covariance (ANCOVA; Fig. 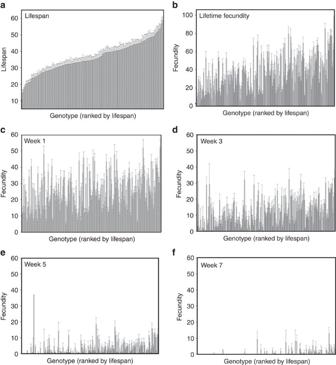Figure 1: Natural genetic variation in mated lifespan, age-specific fecundity and lifetime fecundity. Distribution of line means from 189 measured DGRP lines for (a). Lifespan (n=4,132 females), (b). Lifetime fecundity (n=4,122 females), (c). Week 1 fecundity (n=4,122 females), (d). Week 3 fecundity (n=3,305 females), (e). Week 5 fecundity (n=1,913 females) and (f). Week 7 fecundity (n=684 females). Error bars indicate ±1 s.e.m. We assayed a minimum of 22 females on all lines except six that were difficult to culture (RAL_461, RAL_509, RAL_727, RAL_757, RAL_804 and RAL_832); we assayed 9–17 females of these lines. Sample sizes for each line subsequently decreased with age because females were eliminated from analysis on death. 1 and Table 1 ). Overall, mean fecundity decreased with age ( Supplementary Fig. 1 ). Fecundity differed significantly among lines at all ages ( P <0.0001) as did lifetime fecundity ( χ 2 1 =1343.3, P <0.0001; Supplementary Table 1 ). Although the broad-sense heritability and the genetic variance component ( σ 2 G ) decreased with age ( Table 1 ), when the variance was standardized by the trait mean using the coefficient of variation, CV G [27] , the genetic component of the variation in fecundity increased with age ( Table 1 ). 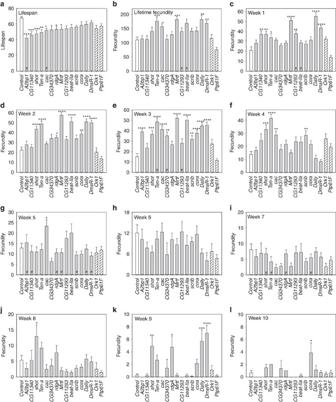Figure 2: Effects of RNAi against candidate genes influencing lifespan and fecundity. Mean phenotype values for (a). Lifespan (n=394 females), (b). Lifetime fecundity (n=391 females) and age-specific fecundity at (c). Week 1 (n=381 females), (d). Week 2 (n=365 females), (e). Week 3 (n=350 females), (f). Week 4 (n=347 females), (g). Week 5 (n=322 females), (h). Week 6 (n=305 females), (i). Week 7 (n=263 females), (j). Week 8 (n=201 females), (k). Week 9 (n=116 females) and (l). Week 10 (n=50 females) for each RNAi line for candidate genes (grey bars) or non-candidate genes (striped bars), and the control line (white bar) crossed with thetubulin-Gal4 driver line. Error bars indicate ±1 s.e.m. Each line began the assay with 30 replicates, and females were eliminated from further analysis on death. RNAi crosses are indicated as significantly different than the control cross at the level of *0.01<P<0.05, **0.001<P<0.01, ***0.0001<P<0.001 or ****P<0.0001 using the Dunnett’s test. Genes that were significant in the DGRP GWA for each age class and trait are demarcated with ‘#’ at the base of the bars. This pattern of increased genetic variance with age also held when we restricted the analysis to include only the 135 lines that survived to week 7 ( Supplementary Table 2 ). There was a significant interaction between line and age ( P <0.0001; Supplementary Table 1 ), indicating that the effect of age on fecundity varied among the DGRP lines ( Supplementary Fig. 1 ). Genetic differences explained 36% of the phenotypic variation in lifetime fecundity ( Table 1 ). We also found significant differences among genotypes in lifespan ( χ 2 1 =988.5, P <0.0001; Supplementary Table 1 ), which explained 29% of the phenotypic variation ( Table 1 ). Figure 1: Natural genetic variation in mated lifespan, age-specific fecundity and lifetime fecundity. Distribution of line means from 189 measured DGRP lines for ( a ). Lifespan ( n =4,132 females), ( b ). Lifetime fecundity ( n =4,122 females), ( c ). Week 1 fecundity ( n =4,122 females), ( d ). Week 3 fecundity ( n =3,305 females), ( e ). Week 5 fecundity ( n =1,913 females) and ( f ). Week 7 fecundity ( n =684 females). Error bars indicate ±1 s.e.m. We assayed a minimum of 22 females on all lines except six that were difficult to culture (RAL_461, RAL_509, RAL_727, RAL_757, RAL_804 and RAL_832); we assayed 9–17 females of these lines. Sample sizes for each line subsequently decreased with age because females were eliminated from analysis on death. Full size image Table 1 Quantitative genetic analysis of mated lifespan and age-specific fecundity. Full size table GWA results We next utilized the DGRP analysis pipeline ( http://dgrp.gnets.ncsu.edu ) to associate variation in our phenotypes with allelic variation at just over 2.49 million SNPs among the DGRP lines using single-marker analysis of variance (ANOVAs) [8] . We identified 1,031 candidate SNPs, within or nearby (less than 5,000 bp away from) 549 putative genes ( Supplementary Data 1 ), affecting fecundity ( P <10 −5 ). The vast majority of these genes were novel associations for fecundity ( Supplementary Data 2 ). Surprisingly, when the data were partitioned by age class, we observed a dramatic increase in the number of SNPs influencing fecundity with increasing age ( Table 2 ). From week 1 to week 3, we observed an 87% increase in the number of SNPs detected, and from week 3 to week 5 we detected 12 times the number of SNPs influencing fecundity. Extending this further, the increase in SNPs detected at 5 weeks was 22 times that of the week 1 analysis. Table 2 Numbers of candidate SNPs and genes associated with fecundity within each age class by GWA at a nominal P <10 −5 . Full size table Several of the 159 total lines used in the GWA did not survive to week 7 and thus were not included in the GWA for fecundity at this age. To ensure that the available sample of alleles in the population did not drastically alter the pattern in our results, we repeated our analysis using only the lines that had survived to week 7. Despite the restricted sample of just 116 genotypes, we still found a drastic increase in candidate SNPs identified in the GWA at late ages compared with early ages. We identified 232 more candidate SNPs in 129 more candidate genes at week 5 compared with weeks 1 and 3 combined. The GWA using all lines showed a 13% decrease in SNPs detected from week 5 to week 7, but this decrease was likely the result of the lowered sample size at week 7. In fact, the restricted analysis using only lines that survived to week 7 revealed another 62% increase in candidate SNPs in the week 7 fecundity GWA as compared to week 5 ( Supplementary Table 2 ). The increase in SNPs with age was consistent across site classes of the candidate SNPs ( Supplementary Table 3 ). There was little linkage among the SNPs that affected age-specific fecundity ( Supplementary Fig. 2 ), increasing the likelihood that these polymorphisms had direct effects on fecundity. The GWA for mated lifespan identified 52 candidate SNPs ( Supplementary Data 1 ) associated with 21 genes that, to the best of our knowledge, were nearly all novel for lifespan ( Supplementary Data 2 ). However, one of our candidates, cacophony (cac) , was recently associated with lifespan in a study examining genetic divergence among control populations and those selected for enhanced late-life reproduction [18] . In addition, seven of our candidate SNPs fall in genomic regions associated with longevity at a 5% false discovery rate threshold in a recent GWA of synthetic Drosophila populations [28] . Genes associated with these SNPs include Cyp6w1 , tRNA:R2:42Aa , CG8343 and Ptr ( Supplementary Data 1 ). Candidate SNPs influencing fecundity are age specific The GWA revealed very little overlap in candidate polymorphisms influencing fecundity between ages or between lifespan and fecundity. Only 23 of the 1,031 fecundity SNPs appeared as candidates in the GWA for two or more of the traits ( Supplementary Table 4 ). A majority of these overlapping SNPs were candidates for fecundity at weeks 1 or 3 and lifetime fecundity (16 SNPs). Given that the lifetime fecundity was largely determined by fecundity at early ages this is not surprising. Five of the remaining SNPs were candidates for both week 5 and week 7 fecundity and only one appeared as a candidate for both early age (week 3) and late age (week 5) fecundity ( Supplementary Table 4 ). Likewise, there was also very little overlap in genes associated with candidate SNPs at each age. Out of 549 genes found to affect fecundity, only 49 genes appeared in more than one age class ( Supplementary Table 4 ). To further verify that the candidate SNPs identified for fecundity were unique to a given age class, we searched for overlaps among the top-ranking SNPs in each age class regardless of significance. We ranked all SNPs assayed by the DGRP analysis pipeline for fecundity at each age (excluding lifetime fecundity) by P -value and compared the top 500 SNPs with the lowest P -value for each age class. We found that 42 SNPs overlapped among the top 500 SNPs between two age classes, and of these, just 13 were among the lowest P -values at early age (weeks 1 or 3) and late age (weeks 5 and 7) ( Supplementary Table 5 ). Functional testing to validate candidate genes To confirm the influence of a subset of our candidate genes on fecundity and/or lifespan, we repeated our age-specific fecundity and lifespan assay using offspring from crosses of 14 candidate UAS–RNAi lines, two non-candidate UAS–RNAi lines ( Ork1, Ptp61F ) and one control line with males of a tubulin -Gal4 line. We chose to validate these genes because the candidate polymorphisms had a variety of age-specific effects on fecundity or lifespan and because there were TRiP RNAi stocks readily available ( http://www.flyrnai.org ). Because the RNAi experiments required measuring far fewer genotypes at a time compared with the mapping experiment with the DGRP, we were able to measure age-specific fecundity every week and we were able to analyse data from older ages. When compared with the control line, all 14 of the candidate genes influenced fecundity at least at one age but the non-candidate genes did not significantly influence fecundity using ANCOVA with a post hoc Dunnett’s test ( Fig. 2c–l ). In addition, none of the candidates significantly affected fecundity at all ages ( Supplementary Fig. 3 ). This finding both validated the influence of these genes on fecundity and confirmed that they can influence fecundity in an age-specific manner. In addition, five of the candidate genes tested with RNAi lines showed an influence on lifetime fecundity ( Fig. 2b ) and seven genes influenced lifespan, two of which were lifespan candidates in our GWA ( Fig. 2a ). The RNAi lines lived substantially longer than the DGRP lines on average (54 versus 36 days). We suspect that this is because the RNAi genotypes were heterozygous and so masked deleterious recessive alleles that would have reduced the average lifespan in the DGRP lines. Figure 2: Effects of RNAi against candidate genes influencing lifespan and fecundity. Mean phenotype values for ( a ). Lifespan ( n =394 females), ( b ). Lifetime fecundity ( n =391 females) and age-specific fecundity at ( c ). Week 1 ( n =381 females), ( d ). Week 2 ( n =365 females), ( e ). Week 3 ( n =350 females), ( f ). Week 4 ( n =347 females), ( g ). Week 5 ( n =322 females), ( h ). Week 6 ( n =305 females), ( i ). Week 7 ( n =263 females), ( j ). Week 8 ( n =201 females), ( k ). Week 9 ( n =116 females) and ( l ). Week 10 ( n =50 females) for each RNAi line for candidate genes (grey bars) or non-candidate genes (striped bars), and the control line (white bar) crossed with the tubulin -Gal4 driver line. Error bars indicate ±1 s.e.m. Each line began the assay with 30 replicates, and females were eliminated from further analysis on death. RNAi crosses are indicated as significantly different than the control cross at the level of *0.01< P <0.05, **0.001< P <0.01, ***0.0001< P <0.001 or **** P <0.0001 using the Dunnett’s test. Genes that were significant in the DGRP GWA for each age class and trait are demarcated with ‘#’ at the base of the bars. Full size image Gene ontology analysis To assess the functional relatedness of our candidates, we completed gene ontology (GO) enrichment analysis using FlyMine [29] . No GO categories were overrepresented based on our lifespan or early-age fecundity (weeks 1 and 3) candidates, but several GO categories were overrepresented among our late-age candidates. GO analysis of our fecundity candidates identified 179 overrepresented Biological Processes GO terms using the Benjamini–Hochberg test and 68 overrepresented GO terms using the more conservative Holm–Bonferroni test, including many terms related to regulation, development, morphogenesis, neural development and function, cellular processes and cell signalling ( Supplementary Data 3 ). Our candidates were also enriched for four and two molecular function GO categories using Benjamini–Hochberg and Holm–Bonferroni tests, respectively. The molecular function categories were related to transcription factor activity and protein binding ( Supplementary Data 3 ). Finally, our candidates were enriched for seven protein domains that are all immunoglobulin or immune-induced proteins ( Supplementary Data 3 ). We used the DGRP to identify polymorphisms underlying the natural variation in lifespan, lifetime fecundity and age-specific fecundity in mated female fruit flies. We found extensive natural genetic variation in all of our phenotypes, and the amount of genetic variation influencing fecundity increased with age. We found minimal overlap in SNPs affecting fecundity between ages: only one SNP was associated with both and early age (weeks 1 or 3) and late age (weeks 5 or 7; Supplementary Table 4 ). Further, the RNAi validation assay showed that despite ubiquitous expression of RNAi against the target candidate gene, the genes tested influenced fecundity in an age-specific manner ( Fig. 2 ). We note that the pattern of age-specific effects of SNPs on fecundity often differed from those of the comparable RNAi experiment. Indeed, the RNAi experiments often found that some genes had effects across more ages than did SNPs in those loci in the mapping experiment with the DGRP lines. Does this then indicate that the SNPs in the mapping experiment do in fact have similar biological affects across age classes, but the DGRP mapping experiment was insufficiently powered to detect this? We do not think this is the case, in part because we actually identified more SNPs affecting fecundity at older ages, despite the fact that fewer lines were laying eggs at older ages and the magnitude of the differences in fecundity among lines was lower at older ages. This should have reduced our power to detect SNPs affecting fecundity at later ages and so reduced the number of SNPs identified. Instead we suggest that the inconsistency between the DGRP mapping results and the RNAi results is due to at least three factors. First, the RNAi lines were constructed in a different genetic background from the DGRP. Thus, epistatic interactions could influence the genetic effects on phenotypes and indeed, epistasis appears to be a pervasive influence on quantitative traits in Drosophila [29] . Second, the flies used in the RNAi experiment were heterozygous, while those in the mapping experiment with the DGRP were inbred. Finally, the tubulin driver we used to drive RNAi expression should reduce expression of the candidate genes ubiquitously in all tissues in the fly. We suspect that natural polymorphisms are likely to have tissue-specific and more subtle effects on phenotypes. In addition, the RNAi experiments also revealed pleiotropic effects of some loci that were not detected in the mapping experiment. This could also be due to the relatively more subtle effects of natural polymorphisms. If so, this would reduce the likelihood of detecting antagonistic pleiotropic loci even if present due to low statistical power to detect them. Future work using larger mapping populations or more targeted experiments focused on identifying pleiotropic effects of candidate polymorphisms are needed to test this idea. Evidence to suggest that the genetic basis of variation in complex traits changes with age has been provided at the levels of QTL [19] , [30] , genes [25] , [31] and transcripts [26] ; however, our work is the first to provide evidence of this at the SNP level. If this is the general case, it suggests that greater insight into the genetic architecture of phenotypic variation will be provided by mapping genotype to phenotype in an age-specific manner. The leading evolutionary theories of senescence are centred around the concept of age-specific allelic effects on fitness. One theory, MA, predicts that deleterious alleles that contribute to variation in senescence can be maintained in a population if they do not influence fitness at early ages. Before our work, support for MA primarily came from studies showing age-related increases in components of genetic variation, the strongest of which came from studies by Charlesworth and Hughes [32] and Hughes et al . [33] , who found an increase in inbreeding load and dominance variance with age, which are unique predictions of MA [34] , [35] . We also observed an increase in genetic variance in fecundity with age, as measured by the CV G ( Table 1 ). Similar increases have been reported for male mating activity [36] , female fecundity [19] , [22] , mating success [32] , [33] and immune function [26] in Drosophila . However, reliance on age-specific components of genetic variation to support evolutionary theories of aging has been criticized because these predictions are only true under certain conditions: constant additive and dominance effects on the phenotype across ages [37] . Genomic approaches (for example, eQTL studies or genome-wide association tests) like ours allow a more direct test of model predictions because the age-specific fitness effects of the polymorphisms themselves can be assessed [38] . The fact that we found a dramatic increase in the number of SNPs affecting fecundity with increasing age and minimal overlap among candidate SNPs across ages ( Table 2 ) provides perhaps some of the strongest support yet for the role of MA in explaining the maintenance of genetic variation in senescence. While many studies have shown that mutations in a variety of genes can influence egg production, very few natural polymorphisms affecting this trait have been identified. One study associated three naturally occurring QTL with early-age fecundity, and these QTL contain several potential candidates affecting this trait ( daughterless, rho-6, zucchini, kekkon-1, vasa, cactus, kelch, maelstrom, jim, rpk, bicoid, poached and squid) [19] . In addition, natural variation in the genes insulin-like receptor [39] , methuselah [40] and Drip [41] have all been associated with natural variation in fecundity. Although the vast majority of the candidate genes identified for fecundity in our study were novel, 61 have previously been associated with some aspect of reproduction, mating or egg development ( Supplementary Data 2 ). In addition, nearly all of our lifespan candidate genes were novel associations for lifespan. However, two of our fecundity candidates, NLaz [42] and Sesn [43] , have previously been associated with lifespan, which suggests that these genes may have pleiotropic effects on these traits. Interestingly, four of our lifespan candidate genes and 63 of our fecundity candidate genes are found in genomic regions that were recently associated with longevity in a GWA that used synthetic recombinant Drosophila populations [28] ( Supplementary Data 1 ). Neuronal signalling is thought to mediate cellular, organ system and whole-body homeostasis in a manner that regulates aging (reviewed in ref. 44 ). Our data support this claim since many of our enriched Biological Processes GO terms were related to neural function or development and signal transduction. In addition, one of our validated candidate genes for lifespan, cac , which codes for the primary α-subunit of presynaptic voltage-gated calcium channels in the Drosophila neural muscular junction [45] , has recently been linked to age-related decreases in synaptic vesicle release probability and presynaptic calcium channel clusters associated with Alzheimer’s disease [46] . The cac gene was also recently associated with divergence in Drosophila populations artificially selected for late-life performance [18] , and its late-age increase in expression was associated with decreased immune function in naturally derived lines [26] . It is increasingly apparent that the genetic architecture of quantitative traits changes with age and moreover that the way that aging influences these traits varies among genotypes. While the mechanism behind this is not clear, there are at least two potential explanations. First, as animals age, physiological changes create different internal environments in which genes and proteins function. Changes in the internal physiological environment then may alter the magnitude of genetic influences on a given trait (in the manner of a genotype by environment interaction). A second possibility is that age-related changes in phenotypes are actively regulated, perhaps through epigenetic mechanisms like histone modification and chromatin remodelling, which have been implicated as major influences on senescence [47] . Genetic variation in age-specific patterns of epigenetic regulation could explain genetically based differences in age-specific traits like fecundity (this study, ref. 19 ) and immunity [26] . Future work to test these ideas is needed to provide a more mechanistic understanding of genetic contributions to senescence. DGRP assay DGRP stocks, provided by Dr Trudy Mackay’s laboratory at North Carolina State University, were maintained at 25 °C and 60% relative humidity under a 12-h light–dark cycle, and were fed a standard molasses/cornmeal/agar diet before experimentation. To minimize maternal effects on experimental results, stocks were constantly maintained at densities of approximately 20 females and 10 males per vial. All stocks were treated with tetracycline [48] at least three generations before experimentation to minimize confounding effects of among-line variation in Wolbachia infection [8] . Wolbachia clearance was verified using PCR amplification of DNA extracts from adult flies of six DGRP lines known to be infected: RAL_362, RAL_365, RAL_555, RAL_705, RAL_707 and RAL_852 (ref. 8 ). DGRP lines RAL_399, RAL_514, RAL_517, known to be uninfected were used as negative controls and the w 1118 laboratory stock was used as a positive control. DNA was extracted using Genomic DNA purification kit (Fermentas), and PCR was completed using PCR master mix (Fermentas) and the primers (IDT) used were wsp 81F (forward): 5′-TGGTCCAATAAGTGATGAAGAAAC-3′ and wsp 691R (reverse): 5′-AAAAATTAAACGCTACTCCA-3′ (ref. 49 ). The PCR programme was 95 °C for 4 min; 35 cycles of 94 °C for 1 min, 50 °C for 1 min, 72 °C for 1 min; 72 °C for 10 min. Electrophoresis revealed Wolbachia infection was successfully cleared in all genotypes tested ( Supplementary Fig. 4 ). To generate experimental flies, 20 females and 10 males from each DGRP line were collected under light CO 2 anaesthesia in 250 ml population bottles capped with small petri dishes containing a 2% agar base painted with ‘larval’ media [23] . After 48 h, plates were removed and larvae were transferred to vials containing 8 ml of larval media at a standardized density of 50 larvae per vial. Newly eclosed virgin females were collected under light CO 2 anaesthesia and immediately transferred to vials containing approximately 4 ml of ‘adult’ media containing 5% sucrose and 5% yeast [23] . These females were maintained as individuals in each vial with a single, age-matched male of DGRP line RAL_774 always present. Flies were transferred to vials containing fresh media at least twice weekly using no anaesthesia. Lifespan was recorded daily and on death, thorax length was measured using an ocular micrometre at × 2.5. This estimate of body size was used as a covariate in statistical analyses. Fecundity was estimated every other week of the female’s lifespan as a 2-day total of eggs laid [19] . Lifetime fecundity was estimated as the sum of all egg counts sampled for each female. We investigated a minimum of 22 mated females for the majority of the 189 DGRP genotypes included in this assay totalling 4,132 flies. Statistical analyses The PROC MIXED procedure in SAS (Version 9.2, SAS Institute, Cary, NC) was used to carry out ANCOVA to detect differences in the phenotypes among lines. Body size, as estimated by thorax length, was evaluated as a covariate in the model and was found to significantly influence all phenotypes except 5- and 7-week fecundity, so it was used as a covariate in the model. Preliminary analysis revealed that the interaction between body size and line was not significant in any model, so the interaction was dropped from the model. We analysed the age-specific fecundity data across ages using the model: y = bs + a + l + b + l * a + ε , where y is the mean 2-day egg count total, bs is the body size (random covariate), a is age (fixed effect), l is the effect of the DGRP line (random effect), b is the effect of block (random effect), l * a is the interaction term between line and age (random effect) and ε is the effect of error. Data from weeks 9 and 11 were excluded from these analyses due to insufficient sample sizes for each line represented. Age-specific fecundity data were analysed within each age using a reduced ANCOVA model: y = bs+l + b + ε with all variables defined as above. Lifetime fecundity and lifespan data were also evaluated using this reduced mixed-model ANCOVA, where y in each model respectively indicates the sum of all 2-day egg totals for a single female or the lifespan in days. Estimates of genetic variance ( σ 2 G ) and environmental variance ( σ 2 E ) for each phenotype were obtained from the ANCOVA output as the among-line and residual variance components, respectively. Phenotypic variance ( σ 2 P ) was calculated as σ 2 P = σ 2 G+ σ 2 E . Broad-sense heritability was calculated as H 2 =( σ 2 G )/( σ 2 P ). Coefficients of genetic variation and environmental variation were calculated as CV G =100√( σ 2 G )/ and CV E =100√( σ 2 E )/, respectively, where indicates the phenotype least squares mean (corrected for body size and block) [27] . To identify candidate SNPs that contribute to variation in our phenotypes, we submitted the least squares line means of each trait (corrected for body size and block) to the DGRP analysis pipeline ( http://dgrp.gnets.ncsu.edu/ ), GWA was completed on 159 of the 189 lines assayed, based on the sequence data available within the pipeline at the time of analysis. The DGRP Freeze 1 Release 5.46 GWA analysis uses simple linear model ANOVAs on approximately 2.49 million SNPs using the model y =μ+ M + ε where M is the effect of the SNP and ε is the error variance [8] . SNPs were only considered if the minor allele was represented by a minimum of four DGRP genotypes in the sample (minimum minor allele frequency was approximately 2% in our case). The output included all candidate SNPs associated with each respective phenotype at a nominal P <10 −5 . In addition, the DGRP output provided information on site class for each SNP: SNPs more than 5,000 base pairs from any known gene were identified as such; SNPs in coding regions were identified as missense, synonymous or nonsense SNP variants, as appropriate [8] . Our first GWA analysis revealed over 2,000 candidate SNPs associated with age-specific fecundity. However, the lines that exhibited the highest fecundity at week 5 (line RAL_356) and week 7 (line RAL_391) were overrepresented with minor alleles in the SNPs identified for those ages. We detected these overrepresentations by totalling the minor alleles at each candidate SNP for each DGRP line in the GWA. The outlier lines had over 1,000 minor alleles, whereas all other lines had less than 400 minor alleles among the candidate SNPs. To decrease the likelihood of identifying false positive associations among our candidates, we dropped these lines from the analysis and re-ran our GWA for weeks 5 and 7. Unless noted otherwise, all data presented here are based on these more conservative analyses. GO information for genes associated with candidate SNPs was obtained from FlyBase version FB2013_01 (ref. 50 ) and FlyMine version 37.0 (ref. 29 ). Candidate gene validation with RNAi stocks To validate the influence of a subset of the candidate genes identified in our GWAS, we used the GAL4/UAS–RNAi system to knockdown the expression of 14 candidate genes for age-specific fecundity or lifespan ( Supplementary Table 6 ). We chose candidate genes that represented associations with fecundity at a variety of ages and lifespan, and that also had RNAi lines available from the Bloomington Drosophila Stock Center ( http://flystocks.bio.indiana.edu ) and created by the Transgenic RNAi Project (TRiP) at Harvard Medical School ( http://www.flyrnai.org ). For consistency, we restricted our candidates to those with RNAi lines available with the attp2 landing site and those with the VALIUM20 or VALIUM10 vector to produce the strongest RNAi effects ( http://www.flyrnai.org ). We also tested two non-candidate genes ( Ork1 ad Ptp61F ) as controls to verify that knocking down gene expression did not universally influence the phenotypes. We crossed females from UAS–RNAi lines with males harbouring the tubulin -Gal4 driver ( Supplementary Table 6 ) to knockdown expression of individual candidate genes in the adult female offspring. The tubulin driver causes ubiquitous RNAi expression against target genes, thus gene expression is knocked down in all tissues and should be knocked down at all ages [51] . We chose this approach as a logical first step in validation of our candidate genes because genes previously associated with fecundity and senescence show increased or decreased expression in different tissues [17] . As such, our intent was to complete this initial screen using ubiquitous expression, and then fine-tune the validated candidates to dissect tissue-specific expression patterns at different ages. We chose to measure fecundity weekly in these flies because differences in the genetic backgrounds of the RNAi lines and the DGRP lines are likely to result in variable rates of reproductive senescence, so sampling fecundity more frequently in this smaller set of lines allows a greater likelihood of capturing the age-specific effects of the focal genes on fecundity. We used the standard control line for TriP RNAi lines with the attp2 landing site ( Supplementary Table 6 ; http://flystocks.bio.indiana.edu , http://www.flyrnai.org ). We measured fecundity weekly and monitored lifespan daily using techniques identical to the DGRP assay described above. To determine which candidate genes had an effect on each trait, we used the reduced mixed-model ANOVA: y = bs+l + b + ε with all variables defined as above followed by post hoc analysis with Dunnett’s test [52] to compare all RNAi lines against the control line. How to cite this article : Durham, M.F. et al . Genome-wide analysis in Drosophila reveals age-specific effects of SNPs on fitness traits. Nat. Commun. 5:4338 doi: 10.1038/ncomms5338 (2014).